Non-polydimethylsiloxane devices for oxygen-free flow lithography Flow lithography has become a powerful particle synthesis technique. Currently, flow lithography relies on the use of polydimethylsiloxane microchannels, because the process requires local inhibition of polymerization, near channel interfaces, via oxygen permeation. The dependence on polydimethylsiloxane devices greatly limits the range of precursor materials that can be processed in flow lithography. Here we present oxygen-free flow lithography via inert fluid-lubrication layers for the synthesis of new classes of complex microparticles. We use an initiated chemical vapour deposition nano-adhesive bonding technique to create non-polydimethylsiloxane-based devices. We successfully synthesize microparticles with a sub-second residence time and demonstrate on-the-fly alteration of particle height. This technique greatly expands the synthesis capabilities of flow lithography, enabling particle synthesis, using water-insoluble monomers, organic solvents, and hydrophobic functional entities such as quantum dots and single-walled carbon nanotubes. As one demonstrative application, we created near-infrared barcoded particles for real-time, label-free detection of target analytes. Liquid-phase particle-synthesis methods have had limited success in creating geometrically and chemically anisotropic particles, owing to the tendency of liquid systems to adopt arrangements that minimize surface energy. In current liquid-based methods, such as batch nucleation [1] , emulsification [2] , microreactor production [3] , droplet-based microfluidics [4] , [5] , droplet template fabrication [6] , [7] , co-jetting [8] , and microcutting [9] , the particle geometries have been restricted to spheres, deformed spheres, or cylinders. Template-assisted particle fabrication [10] , [11] , [12] , [13] has been developed for the creation of geometrically complex particles with sub-micrometer dimensions. However, this method is largely ineffective at producing particles with chemical anisotropy or patterning, as the precursor liquid is simply isolated in a non-wetting template and then crosslinked in situ . Although one-dimensional striped particles have been generated [14] , the synthesis requires complex steps including multiple evaporation-refilling-crosslinking procedures, and the process cannot be applied to nonvolatile precursors. Microfluidic methods provide a flexible toolset for patterning precursor liquids in the synthesis process. The low Reynolds number regime of microfluidic devices offers several advantages that can be exploited for the generation of nano- and micro-particles [15] , [16] . Complex laminar flow patterns can easily be established in microfluidic channels without the need for physical separators, enabling a range of applications that cannot be achieved with more traditional liquid-handling technologies [17] , [18] , [19] , [20] . Flow lithography (FL) is a versatile technique that combines photolithography with the capabilities of microfluidic methods, for the high-fidelity synthesis of a wide range of complex gel microparticles [21] , [22] , [23] , [24] . In this technique, photomask-defined shapes can be rapidly printed onto structured micro-flows, providing precise control over particle size, geometry, and chemical patchiness. FL has been used extensively for the preparation of multifunctional particles with applications in diagnostics [25] , [26] , [27] assembly [28] , microelectromechanical systems [29] , [30] , photonics [31] , and tissue engineering [32] . Current FL protocols require polydimethylsiloxane (PDMS) channels to allow for the permeation of oxygen into the synthesis chamber for inhibition of polymerization near channel interfaces. This localized inhibition layer enables the production of mobile particulates (as opposed to fixed structures) that can be transported out of the synthesis area via flow [22] . The current dependence on PDMS places restrictions on both device construction (for example, glass or plastic cannot be used) and prevents the use of solvents and/or monomers that swell PDMS. Employing an initiated chemical vapour deposition (iCVD) nano-adhesive bonding procedure, to construct a new class of non-PDMS devices, we now present oxygen-free FL, a versatile particle-synthesis method that uses inert fluid-lubrication layers to achieve new levels of chemical complexity. By vertically layering multiple laminar flows within this new generation of devices, we produce anisotropic particles, using sub-second residence times without oxygen-lubrication layers, and tune particle heights on demand by adjusting flow parameters. We further estimate maximum residence time for particle synthesis, evaluating physical and kinetic properties such as flow layer thickness, critical gel point, and diffusivity. Finally, we demonstrate solvent-based synthesis of complex anisotropic particles from structured microflows of water-insoluble monomers and particles encapsulating hydrophobic functional entities such as ruthenium, quantum dots (QDs) and single-walled carbon nanotubes (SWNTs). Using this approach, we synthesize graphically encoded particles that bear near-infrared (NIR)-active QDs in the 'code' region and SWNTs in a separate 'probe' region designed for label-free, real-time detection of target molecules. The novel techniques, described here, greatly enhance the synthesis capabilities of FL and further expand the library of chemically and geometrically complex microparticles that can be produced. iCVD nano-adhesive bonding to fabricate non-PDMS-based devices Oxygen-free FL is a technique designed to extend current PDMS-based FL to non-PDMS-based devices. These non-PDMS-based devices include homogeneous and heterogeneous devices created from numerous combinations of alternative substrate materials, as well as integrated devices, to mount electric and magnetic circuits. In past work, the absence of a suitably general bonding method to combine diverse types of substrates has led to limitations in device construction. In developing oxygen-free FL, we required a bonding method that does not depend on substrate type for the creation of a wide array of devices with different properties, does not demand immediate bonding for further device integration, and offers strong mechanical resistance for high-throughput synthesis. With these considerations in mind, we use the nano-adhesive iCVD-bonding technique for the creation of non-PDMS-based devices. The versatile iCVD method is able to deposit conformal and pinhole-free adhesive films on virtually any kind of substrate with nanometer-level thickness control [33] , [34] , [35] . Also, the iCVD-bonding process is independent of the channel fabrication process, and deposited samples can be stored for more than 2 months before bonding [34] , [35] . Finally, bonded devices were able to withstand pressures higher than 150 psia, and the all-iCVD nano-adhesive bonding process showed superior resistance against hydrolytic degradation [35] . We demonstrate that the iCVD nano-adhesive bonding technique can be used to fabricate non-PDMS-based channels. Ultraviolet-curable Norland Optical Adhesive 81 (NOA81), a thiolene-based resin, was chosen as the substrate material ( Supplementary Figs S1 and S2 ), because it is commercially available and allows for rapid prototyping and reliable replication of sub-micron features [36] . In addition, this material can provide a number of attractive optical and physical properties including transparency, high elastic modulus ( ∼ 3 GPa), and excellent solvent resistance [36] . A nano-adhesive bonding process, utilizing iCVD, has been developed previously [34] , [35] . However, in the past construction of such devices, one substrate was required to be a soft elastic PDMS substrate to ensure conformal contact to the other substrate [34] , [35] . When hard channel substrates were combined together, air bubbles were entrapped between channel interfaces, causing insufficient channel sealing and even distortion of channel geometries. To overcome this, we developed a vacuum-curing process to remove the trapped air bubbles and, for the first time, generated homogeneous NOA81 channels using the bonding technique ( Fig. 1a ). It should be noted that the NOA81 channels can also be prepared by existing thiolene-based bonding techniques [36] , [37] , [38] . However, these existing methods do not satisfy all of the previously mentioned requirements for oxygen-free FL, thereby limiting operational flexibility. We further demonstrated that the iCVD nano-adhesive bonding technique can be used to construct heterogeneous NOA81channels ( Supplementary Fig. S3 ). 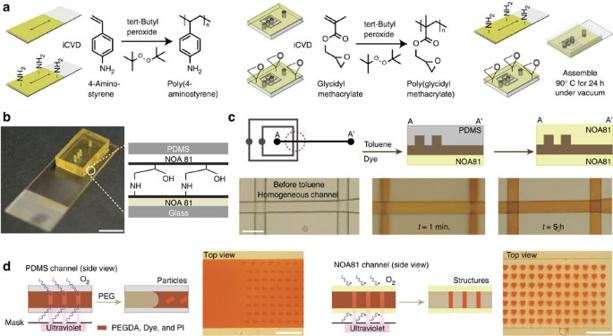Figure 1: iCVD nano-adhesive bonding. (a) Schematic description of the conformal iCVD nano-adhesive bonding process. The process is described in detail in the Methods Section. (b) Colour image of fully assembled channel mounted on a glass slide. The inserted schematic describes the bonding chemistry between channel interfaces. (c) Comparison of hybrid PDMS-Norland optical adhesive (NOA) and homogeneous NOA channels for solvent resistance. Using a ×20 objective indicated by the dashed red circle in the schematic, we examined the area highlighted in images. The organic solvent was seen to swell and significantly deform the channel segments constructed from PDMS after only 1 min of exposure in the hybrid device, while the homogeneous NOA device maintained its integrity even after 5 h of exposure. (d) Comparison of homogeneous PDMS and NOA channels for ultraviolet-initiated FL using mask template. PDMS channels allow for oxygen permeation, which terminates polymerization at the top and bottom faces of the device and thereby enables the creation of microparticles that can be removed via flow. In contrast, gas-impermeable NOA channels do not produce such a lubricating layer, thus creating structures fixed to the surfaces of the channel. Monomer solution consists of PEGDA 700, red acrylate 13, and PI whereas rinse solution is pure PEG 200. Scale bars, (b) 1 cm, (c) 80 μm, and (d) 100 μm. Figure 1: iCVD nano-adhesive bonding. ( a ) Schematic description of the conformal iCVD nano-adhesive bonding process. The process is described in detail in the Methods Section. ( b ) Colour image of fully assembled channel mounted on a glass slide. The inserted schematic describes the bonding chemistry between channel interfaces. ( c ) Comparison of hybrid PDMS-Norland optical adhesive (NOA) and homogeneous NOA channels for solvent resistance. Using a ×20 objective indicated by the dashed red circle in the schematic, we examined the area highlighted in images. The organic solvent was seen to swell and significantly deform the channel segments constructed from PDMS after only 1 min of exposure in the hybrid device, while the homogeneous NOA device maintained its integrity even after 5 h of exposure. ( d ) Comparison of homogeneous PDMS and NOA channels for ultraviolet-initiated FL using mask template. PDMS channels allow for oxygen permeation, which terminates polymerization at the top and bottom faces of the device and thereby enables the creation of microparticles that can be removed via flow. In contrast, gas-impermeable NOA channels do not produce such a lubricating layer, thus creating structures fixed to the surfaces of the channel. Monomer solution consists of PEGDA 700, red acrylate 13, and PI whereas rinse solution is pure PEG 200. Scale bars, ( b ) 1 cm, ( c ) 80 μm, and ( d ) 100 μm. Full size image The nano-adhesive bonding process was able to combine channel substrates, as well as to retain a range of substrate properties. The NOA devices bonded with the nano-adhesive were optically transparent, compatible with standard photolithography techniques, and showed response time characteristics far superior to those of PDMS channels ( Fig. 1b , Supplementary Note 1 ) [35] , [36] . Also, the devices exhibited excellent compatibility with organic solvent flows, with little evidence of swelling or deformation in numerous trials ( Fig. 1c ; Supplementary Movie 1 ). To demonstrate the improvement over previous iCVD nano-adhesive work [34] , [35] , we first fabricated a two-layer hybrid channel (PDMS top, NOA81 bottom) and injected toluene at the inlet of the bottom channel. When the toluene reached the PDMS substrate, the PDMS channels began to shrink dramatically, and within 1 min, the width of the top PDMS channel was reduced by ∼ 60%. The reduction of channel size can significantly alter flow rates and velocity profiles, and thus prevent the creation of stable layered flows. We then performed the same experiments with homogeneous NOA81 channels and examined their performance with organic solvent flows. Unlike the hybrid channels, we observed no significant swelling, even after 5 h of solvent exposure. This is the first demonstration that the devices bonded by the nano-adhesive technique have solvent resistance. Lastly, as NOA81 substrates are gas-impermeable, the devices cannot provide oxygen-lubrication layers for the creation of free-floating particles ( Fig. 1d ). On-the-fly particle synthesis with sub-second residence time Oxygen-free FL is a technique developed to eliminate the requirement for oxygen lubrication in the FL process by utilizing inert flows that cannot propagate the polymerization reaction ( Supplementary Movie 2 ). Combining a hydrodynamic flow-focusing technique with a compressed-air-flow control system [24] , [39] , we generated pulsed tri-layered flows containing two bounding inert flows and a central monomer flow ( Fig. 2a ; Supplementary Fig. S4 ). Although vertical flow-focusing techniques have been used in flow cytometry [40] , [41] , this is the first demonstration of particle synthesis with stacked lubrication layers. Moreover, it is important to note that our synthesis with the stacked lubrication layers was achieved with a pulsed flow regime that periodically stopped the flow just before the photopolymerization step to provide higher feature resolution and improved throughput ( Supplementary Note 2 and Supplementary Table S1 ) [22] . As pressure-driven sources typically provide quick dynamic response [39] , [42] , we generated rapid pulsing of the layered microflows using our pressure-control system that can allow for fast and simple modulation [39] . We rapidly polymerized cylindrical particles in the middle monomer layer by terminating the driving pressure, waiting 300 ms to ensure complete flow stoppage, and then exposing the flow to a 75-ms ultraviolet burst. We then re-initiated pressure-driven flow for 1 s to flush particles out to the reservoir ( Fig. 2a ). This process was cycled and automated using a computer-controlled system. There were three main criteria for the inert flows: miscibility with the middle monomer to avoid interfacial tension, similar density with the middle monomer to prevent gravity-induced reorientation of interfaces [43] , and a concentration of photoinitiator (PI) that matched the concentration contained in the middle monomer to ensure homogenous polymerization. To satisfy these conditions, we used polyethylene glycol (PEG) with PI for the inert flows for synthesis trials with a central monomer of polyethylene glycol diacrylate (PEGDA). 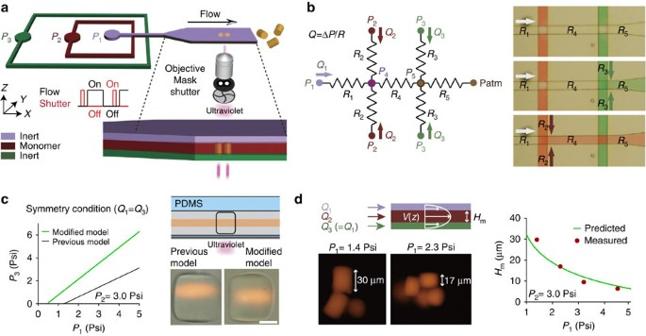Figure 2: On-the-fly alteration of particle height with inert flows. (a) Schematic of microparticle synthesis in gas-impermeable NOA channel. Particles were synthesized and then carried out of the synthesis area using rapid, synchronized cycles of shutter-mediated ultraviolet exposure and pressure-driven flow. The vertical flow focusing process is precisely described inSupplementary Fig. S4. (b) Modified hydrodynamic resistance model used to determine hydrodynamic resistances of various segments of synthesis channel and to estimate volumetric flow rates from inlet pressures. We created three specific hydrodynamic cases:Q1≠0,Q2,Q3=0 (Top),Q1,Q3≠0,Q2=0 (Middle), andQ1,Q2≠0,Q3=0 (Bottom). We then measured inlet pressures that satisfied each case and generated a resistance diagram to extract hydrodynamic resistances (Supplementary Fig. S6). The process is explained in detail in the Methods Section. (c) Comparing modified hydrodynamic model with the previous model in achieving the symmetry condition (Q1=Q3). To visualize the symmetrical inert layers, three-layered particles were synthesized in a PDMS channel. WhenP2was fixed to 3.0 psi,P3satisfying the symmetry condition at a specificP1(=4.9 psi) was predicted from each model. Symmetrical particles were prepared by the use of inlet pressures predicted from the modified model. (d) Particle height as a function ofP1. Height of cylindrical particles was seen to vary with inlet pressures in a manner that matched predictions from the hydrodynamic resistance model. As shown in the graph, theHmprediction compared well with measurements of particle heights. Scale bar, 10 μm. Figure 2: On-the-fly alteration of particle height with inert flows. ( a ) Schematic of microparticle synthesis in gas-impermeable NOA channel. Particles were synthesized and then carried out of the synthesis area using rapid, synchronized cycles of shutter-mediated ultraviolet exposure and pressure-driven flow. The vertical flow focusing process is precisely described in Supplementary Fig. S4 . ( b ) Modified hydrodynamic resistance model used to determine hydrodynamic resistances of various segments of synthesis channel and to estimate volumetric flow rates from inlet pressures. We created three specific hydrodynamic cases: Q 1 ≠0, Q 2 , Q 3 =0 (Top), Q 1 , Q 3 ≠0, Q 2 =0 (Middle), and Q 1 , Q 2 ≠0, Q 3 =0 (Bottom). We then measured inlet pressures that satisfied each case and generated a resistance diagram to extract hydrodynamic resistances ( Supplementary Fig. S6 ). The process is explained in detail in the Methods Section. ( c ) Comparing modified hydrodynamic model with the previous model in achieving the symmetry condition ( Q 1 = Q 3 ). To visualize the symmetrical inert layers, three-layered particles were synthesized in a PDMS channel. When P 2 was fixed to 3.0 psi, P 3 satisfying the symmetry condition at a specific P 1 (=4.9 psi) was predicted from each model. Symmetrical particles were prepared by the use of inlet pressures predicted from the modified model. ( d ) Particle height as a function of P 1 . Height of cylindrical particles was seen to vary with inlet pressures in a manner that matched predictions from the hydrodynamic resistance model. As shown in the graph, the H m prediction compared well with measurements of particle heights. Scale bar, 10 μm. Full size image We developed a predictive model for the creation of particles with inert flows that allowed us to adjust particle height in a systematic fashion. In this approach, the volumetric flow rates for the top and bottom inert flows were designed to be equal to give symmetrical inert thickness in the synthesis chamber. To estimate volumetric flow rates from the measured inlet driving pressures, we previously developed a model that calculated hydrodynamic resistances from channel geometries ( Supplementary Fig. S5; Supplementary Table S2 ) and fluid viscosities [24] . However, this model neglected resistances that arose from inlets, corners, defects and misalignments. To address this, we created a modified model that experimentally determined total hydrodynamic resistances by lumping previously neglected factors ( Fig. 2b , Supplementary Fig. S6 ). Using the estimated hydrodynamic resistances for each channel segment ( Supplementary Table S3-S6 ), we were able to determine inlet pressure relations that provided the desired symmetry condition ( Q 1 = Q 3 ) ( Supplementary Note 3 ). Experimental results validated that the modified model could provide accurate predictions for the inlet pressures required to generate symmetrical inert flows ( Fig. 2c ). Using the symmetry condition, we were able to predict the thickness of the middle monomer layer ( H m ) from the following mass conservation and Poiseuille flow velocity profile for our slit-like channels: where B is the ratio of the volumetric flow rates of inert flow ( Q 1 ) divided by the volumetric flow rate of the middle monomer flow ( Q 2 ), ρ is the density of flow, v is the velocity of flow, h c is channel half-height, and h m is half of the middle flow layer thickness. Solving these equations ( Supplementary Note 4 , Supplementary Fig. S7 ), the analytical expression for H m is: Estimating the flow time to the synthesis zone to be <200 ms, the overall monomer residence time (flow time+stop time+polymerization time) was ∼ 500 ms, which was much smaller than the characteristic time to diffuse the channel height ( h c 2 / D PEGDA575 ∼ 80 s, Fig. 3b ). As a result, the particle heights could be taken to be the same as the middle layer thickness without considering the additional contribution by monomer diffusion. By rationally adjusting inlet pressures, oxygen-free FL can be used to rapidly vary particle height in a channel with a fixed height ( Fig. 2d ; Supplementary Fig. S8 ). Current FL can synthesize only one particle height from any given device, as the oxygen inhibition layer thickness is fixed to ∼ 2 μm, and, thus, new master molds and PDMS devices must be prepared for each different particle height that is desired, a time- and labor-intensive process. In our current set-up, the smallest particle height that we achieved was ∼ 3 μm, which was near the theoretical limit ( ∼ 2 μm, Supplementary Note 5 ). 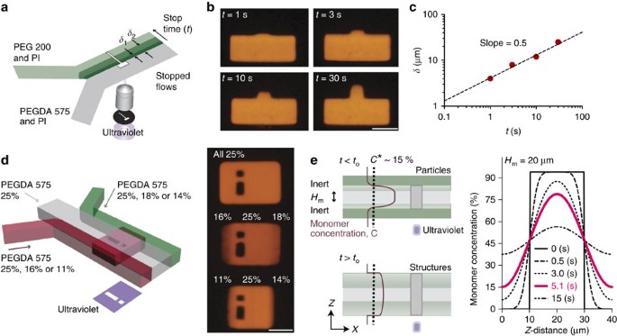Figure 3: Optimization of residence timescale. (a) Experimental set-up for measurement of diffusion coefficient of PEGDA 575 in PEG 200 in a PDMS device. The green stream consists of PEG 200 90% (v/v), PI 5% (v/v), food colouring 4% (v/v), and rhodamine acrylate 1% (v/v), while the grey stream is consisted of PEGDA 575 94% (v/v), PI 5% (v/v), and rhodamine acrylate 1% (v/v). 'T'-shaped exposure mask was used to determine the penetration depth (δ) of PEGDA. (b) Fluorescence images of particles produced with various residence times. (c) Penetration depth as a function of residence time. (d) Variation of PEGDA 575 loading percentage to determine critical gel point (∼15% monomer concentration). Synthesis was performed in PDMS devices, and all streams contained rhodamine acrylate for visualization of particle interfaces. (e) Diffusion model for determination of time,t0, at which critical gel point front reaches walls of gas-impermeable device and induces particle sticking. Simulation solution indicates the maximum residence time is 5.1 s for the creation of particles atHm=20 μm. Scale bars, (b) 50 μm and (d) 40 μm. Figure 3: Optimization of residence timescale. ( a ) Experimental set-up for measurement of diffusion coefficient of PEGDA 575 in PEG 200 in a PDMS device. The green stream consists of PEG 200 90% (v/v), PI 5% (v/v), food colouring 4% (v/v), and rhodamine acrylate 1% (v/v), while the grey stream is consisted of PEGDA 575 94% (v/v), PI 5% (v/v), and rhodamine acrylate 1% (v/v). 'T'-shaped exposure mask was used to determine the penetration depth ( δ ) of PEGDA. ( b ) Fluorescence images of particles produced with various residence times. ( c ) Penetration depth as a function of residence time. ( d ) Variation of PEGDA 575 loading percentage to determine critical gel point ( ∼ 15% monomer concentration). Synthesis was performed in PDMS devices, and all streams contained rhodamine acrylate for visualization of particle interfaces. ( e ) Diffusion model for determination of time, t 0 , at which critical gel point front reaches walls of gas-impermeable device and induces particle sticking. Simulation solution indicates the maximum residence time is 5.1 s for the creation of particles at H m =20 μm. Scale bars, ( b ) 50 μm and ( d ) 40 μm. Full size image Estimation of maximum residence timescale In the synthesis of particles using inert lubrication layers, a short residence time is desirable to minimize the monomer/species diffusion into inert flows. However, complex particles that are generated by applying gravitational, magnetic or electrical fields often require longer residence times, so that the external field can act sufficiently on the system. For example, structurally coloured particles are typically prepared with a residence time >1 s to tune one-dimensional photonic crystal colours by magnetic field modulation and to fix the colour with localized ultraviolet exposure [26] . To investigate transverse diffusion of monomer and the suitability of our strategy for longer residence times, we designed an experiment to visualize the diffusional thickness of PEGDA 575 in PEG 200 ( Fig. 3a ). In this experiment, we used PDMS channels to generate co-flows with a simple two-dimensional flow-focusing technique. One of the co-flows was a green inert flow while the other was a grey monomer flow. We stopped the flow for specified amounts of time to allow monomer to diffuse into the inert flow. Then, we synthesized 'T'-shaped particles at the fluid interface such that the head of the 'T' was aligned with the interface and the leg of the 'T' could be used as an indicator of monomer penetration length ( δ ). Because the stop time was much larger than the sum of the flow and exposure times ( ∼ 100 ms), we assumed the residence time to be roughly equal to the stop time. As shown in Fig. 3b , the diffusion length increased when the residence time was increased, and the value of the slope (0.5) in a log–log plot of diffusional thickness ( δ ) versus residence time ( t ) confirmed the diffusion-based transport ( Fig. 3c ). To extract the diffusion coefficient of PEGDA 575 from the measured diffusion length, we determined the critical gel point of the monomer ( ∼ 15%) by visually checking for gelation at various monomer concentrations ( Fig. 3d ) and applied this to the one-dimensional transient diffusion model. This yielded a diffusivity of 5 μm 2 s −1 , which compared favourably with the value (7 μm 2 s −1 ) calculated from the combination of the literature [44] and the Stokes–Einstein equation ( Supplementary Note 6 ; Supplementary Table S7 ). We then returned to the layered flow system of the gas-impermeable devices and, again assuming one-dimensional transient diffusion, found the following analytical solution for the evolution of monomer concentration in the z -direction ( Supplementary Note 7 ). where C 0 is the initial concentration of monomer in the middle layer, η is the non-dimensionalized z coordinate, and τ is the non-dimensionalized time coordinate. This solution could then be used to determine the maximum residence time, t 0 , at which the critical gel point front reaches the walls of the device and induces particle sticking. For typical synthesis conditions ( h m =20 μm, C 0 =95%), t 0 is ∼ 5.1 s, indicating an operating window that could potentially be exploited in the future for the creation of particles with added complexity. In addition, an accompanying COMSOL simulation showed good agreement with the maximum residence time calculated from the analytical solution ( Fig. 3e ; Supplementary Fig. S9 ). Oxygen-free FL with organic precursors Perhaps the most valuable feature of the oxygen-free FL in NOA devices is the ability to synthesize anisotropic particles using organic solvents, a process that is not possible with current PDMS-based FL approaches. We demonstrated the synthesis of anisotropic particles encapsulating ruthenium complex (II) dyes dispersed in methanol/toluene (4:1 v/v) mixture ( Fig. 4a ). Previous work has shown that encapsulated ruthenium dyes in PEG structures can be used for oxygen-sensing applications [45] , [46] . Furthermore, particle-based sensors offer several detection advantages over microarrays and similar arrangements of immobile structures, including faster capture kinetics and rapid probe-set modification for more flexible assays [26] , [27] . For this study with NOA81 devices and inert flows, we successfully synthesized triangular particles that exhibited homogeneous fluorescent signal, thus confirming entrapment of the ruthenium dyes ( Fig. 4b,c ). This proved that the new FL process could encapsulate functional entities inside particles with the same spatial resolution and efficacy as prior methods. 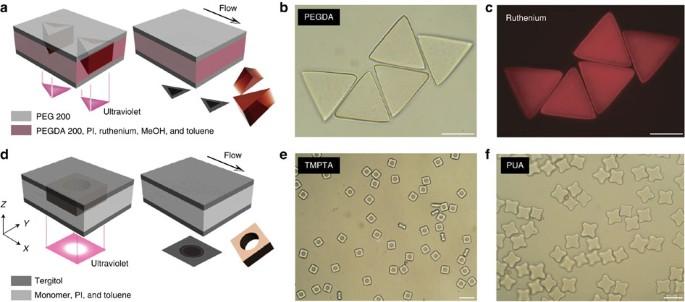Figure 4: Anisotropic particle synthesis from organic precursors. (a) Triangular particle synthesis with PEG 200 inert flows in an NOA channel from organic precursor containing PEGDA 200, ruthenium dye (mixed with methanol (MeOH) and toluene), and PI. (b,c) Brightfield and fluorescence images of triangular particles synthesized in (a). (d) Particle synthesis in an NOA device with water-insoluble monomers TMPTA and PUA, mixed with toluene and PI. Inert flows consisted of Tergitol surfactant to lower surface energy and prevent curvature in top and bottom faces of particle. (e,f) Images of particles synthesized from TMPTA and PUA. Scale bars, (b,c) 30 μm, (e) 100 μm, and (f) 50 μm. Figure 4: Anisotropic particle synthesis from organic precursors. ( a ) Triangular particle synthesis with PEG 200 inert flows in an NOA channel from organic precursor containing PEGDA 200, ruthenium dye (mixed with methanol (MeOH) and toluene), and PI. ( b , c ) Brightfield and fluorescence images of triangular particles synthesized in ( a ). ( d ) Particle synthesis in an NOA device with water-insoluble monomers TMPTA and PUA, mixed with toluene and PI. Inert flows consisted of Tergitol surfactant to lower surface energy and prevent curvature in top and bottom faces of particle. ( e , f ) Images of particles synthesized from TMPTA and PUA. Scale bars, ( b , c ) 30 μm, ( e ) 100 μm, and ( f ) 50 μm. Full size image We also synthesized geometrically complex particles from water-insoluble monomers dissolved in toluene ( Fig. 4d ). We chose to demonstrate this capability with TMPTA (Trimethylolpropane triacrylate, ρ =1.06 g ml −1 ) and PUA (Polyurethane acrylate, ρ =1.09 g ml −1 ), water-insoluble monomers with applications in particle assembly [47] and soft molding [48] , respectively. We could easily modulate the monomer composition in toluene to tune both chemical and mechanical properties of the microparticles. In this hydrophobic monomer system, we replaced the previously used PEG 200 inert flows with tergitol NP-10 ( ρ =1.06 g ml −1 ), because the hydrophilic PEG was immiscible with the monomers and produced curved particle surfaces. The amphiphilic tergitol surfactant had good miscibility with and the same density as the monomers selected. In tri-layered tergitol-monomer-tergitol flows, we successfully created TMPTA and PUA particles using two different mask shapes ( Fig. 4e,f ). The generated particles were optically transparent and rigid enough to allow for rinsing in organic solvents without swelling-based deformation. Synthesis of near-infrared-active anisotropic particles To further demonstrate the utility of oxygen-free FL, we synthesized NIR-active anisotropic particles from organic precursors. NIR fluorescence is emitted in a 'biologically transparent' window, thereby minimizing auto-fluorescence interference and tissue scattering [49] . Through the use of organic precursors that contain NIR-active nano-entities, we introduce unprecedented shape-encoded and barcoded particles that exhibit NIR fluorescence around the NIR II region (wavelengths between 1 ∼ 1.4 μm) to maximize light penetration depth in tissue [50] . NIR-active QDs are more easily prepared in organic solvents than in water, because the former provide synthetic advantages for the production of narrow size distributions as well as a wide range of available sizes [51] . The highest quality QDs produced from organic solvents are both hydrophobic and water-insoluble, making them incompatible with former FL techniques. We purchased commercial hydrophobic QDs dispersed in toluene and bearing a CdTeSe/ZnS core-shell structure with a NIR 915-nm emission peak. To ensure high trapping efficiency of the small QDs (1–10 nm) within the polymer matrix, we used NOA81 instead of PEGDA. Although the minimum pore size of our PEG system can reach ∼ 1 nm (ref. 52 ), PEG hydrogel particles can swell in water, leading to leakage of physically encapsulated QDs, a process that could introduce serious toxicity issues for potential biological applications. NOA81 is biocompatible [36] and has smaller pores, which prevents the loss of entrapped QDs. To evenly disperse QDs in NOA81, we mixed the monomer with a QD solution at a 1:1 volume ratio. Then, we placed the resulting mixture layer between inert tergitol layers and produced triangular particles. The particles physically encapsulated QDs, as shown by the strong NIR photoluminescence (PL) signals in Fig. 5a . Next, we synthesized particles with different loading concentrations of QDs and quantified the PL intensities exhibited by each batch. As expected, we found a simple linear relation between loading concentration and PL intensity ( Fig. 5b ). 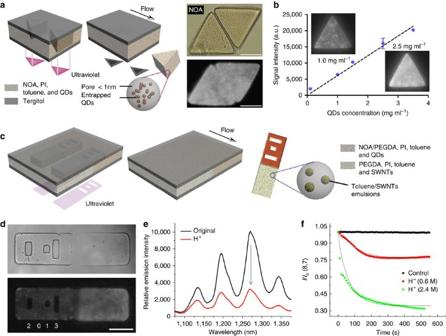Figure 5: Synthesis of NIR-active anisotropic particles. (a) NIR-active triangular particle synthesis. NIR emitting CdTeSe/ZnS QDs were physically entrapped in NOA polymer particles produced in an NOA device. (b) Fluorescent signal intensity as a function of quantum dot loading concentration. Fluorescence was integrated over a circle of radius 30 μm centred on the triangular particles. Each point represents mean measurement from three particles; error bars represent standard deviation. (c) NIR-active multifunctional encoded particle synthesis. Using Tergitol for inert flows, Janus particles were created with a graphical barcode bearing NIR emitting QDs and a separate probe region embedded with single-walled nanotubes (SWNTs) for label-free H+detection. The structured microflows were prepared by the process described inSupplementary Fig. S10. (d) DIC and NIR photoluminescence images of particles from (c). (e) Shift in emission spectrum of embedded SWNTs on introduction of 2.4 M HCl. Blue arrow indicates most pronounced shift, produced by (8,7)-type SWNT. (f) Intensity decay for (8,7)-type SWNT during H+detection. Exponential quenching model was fit to the experimental data, providing moderate proton quenching kinetic parameters of 0.01 and 0.02 s−1for 0.6 and 2.4 M, respectively. All scale bars, 50 μm. Figure 5: Synthesis of NIR-active anisotropic particles. ( a ) NIR-active triangular particle synthesis. NIR emitting CdTeSe/ZnS QDs were physically entrapped in NOA polymer particles produced in an NOA device. ( b ) Fluorescent signal intensity as a function of quantum dot loading concentration. Fluorescence was integrated over a circle of radius 30 μm centred on the triangular particles. Each point represents mean measurement from three particles; error bars represent standard deviation. ( c ) NIR-active multifunctional encoded particle synthesis. Using Tergitol for inert flows, Janus particles were created with a graphical barcode bearing NIR emitting QDs and a separate probe region embedded with single-walled nanotubes (SWNTs) for label-free H + detection. The structured microflows were prepared by the process described in Supplementary Fig. S10 . ( d ) DIC and NIR photoluminescence images of particles from ( c ). ( e ) Shift in emission spectrum of embedded SWNTs on introduction of 2.4 M HCl. Blue arrow indicates most pronounced shift, produced by (8,7)-type SWNT. ( f ) Intensity decay for (8,7)-type SWNT during H + detection. Exponential quenching model was fit to the experimental data, providing moderate proton quenching kinetic parameters of 0.01 and 0.02 s −1 for 0.6 and 2.4 M, respectively. All scale bars, 50 μm. Full size image Of particular interest, we fabricated NIR-barcoded particles embedded with QDs in the code region and SWNTs in the probe region using tri-layered microflows that contain two bounding inert flows and two distinct monomers in the central flow layer ( Fig. 5c; Supplementary Fig. S10 ). The central stream corresponding to the code was the same composition as the previous QD monomer mixture, except 20% (v/v) of toluene was replaced with PEGDA 700 to promote gelation at the probe/code interface. The central stream corresponding to the probe was PEGDA/PI containing 30% (v/v) SWNTs/toluene dispersion. Dispersing SWNTs in the PEGDA/PI mixture presented a significant challenge due to the SWNTs tendency to aggregate in the meta-phase of the hydrophilic monomer and hydrophobic PI. Although SWNTs can be dispersed via covalent attachment of a polymer to their sidewall, this covalent functionalization disrupts the electronic structure and PL of the SWNT [53] , [54] . Therefore, it is crucial to stably disperse SWNTs with polymers in a non-covalent manner to retain the properties that make them effective optical sensors [55] . To overcome these difficulties, we non-covalently dispersed SWNTs by hydrophobic poly(9,9-di-n-dodecylfluorenyl-2,7-diyl) polymer (PDDF) in toluene to preserve their sensing abilities. Then, we mixed the solution with PEGDA/PI by vortexing for 30 s and dispersed SWNTs in the monomer mixture by toluene solvation. By sandwiching the two central streams between bounding tergitol flows, we were able to synthesize bifunctional barcoded particles. In NIR imaging of the particles, we observed the expected signal patterns from the '2013' graphical code region and the SWNT-embedded probe region ( Fig. 5d ). Importantly, the NIR fluorescence of barcoded particles was stable during long periods of laser excitation, a feature that is crucial for read-out of barcodes and accurate quantification of targets in real-time experiments. The SWNTs embedded within probe regions were able to detect a specific target in real-time, with label-free reporting of the binding events. Selectivity for a particular target was achieved by adjusting the wrapping of compounds around the SWNTs [55] , [56] . This ability to tune selectivity suggests that this platform can be used for the multiplexed detection of several targets in a single assay. A distinct advantage of the SWNT probes used in these experiments is the possibility of label-free detection. When a SWNT encounters a target, the PL signal intensity of the SWNT is reduced and the emission wavelength shifts. This emission change allows for the detection and quantification of targets without complex post-target-capture labelling steps, thereby streamlining the assay process and eliminating the possibility of cross-reactivity between probes and labelling reagents. To illustrate the sensing capabilities of NIR fluorescence-barcoded particles, we performed simple proton detection through NIR-fluorescence response. Before the introduction of protons, the spectrum of the probe region showed peaks generated from different types of SWNTs: (9,2), (11,3), (8,7) and (12,4). Among the four peak signals, we used the highest signal of (8,7) type for the analysis. On the introduction of 2.4 M HCl, the signal of (8,7) type was reduced to 26% of the original signal ( Fig. 5e ). We also extracted proton quenching kinetic information, as the signal reduction was tracked in real-time. We used an exponential quenching model to fit experimental data and found quenching kinetic parameters of 0.01 and 0.02 s −1 for 0.6 and 2.4 M target concentrations, respectively ( Fig. 5f ). Oxygen-free FL greatly expands the synthesis capabilities of FL in the following three categories: device construction, process control, and operable material. The new technique can be used in virtually any type of device, whereas conventional FL techniques have been limited to PDMS devices. To achieve this flexibility, we utilized the iCVD nanoadhesive-bonding technique for device construction. This strong and highly flexible bonding method greatly augments the range of devices that can be used, which in turn provides a variety of unique environments for particle synthesis. For example, the synthesis, described here, with the iCVD nano-adhesive and inert flows could be integrated with indium tin oxide substrate, for the fabrication of three-dimensional photonic crystal particles via dynamic modulation of electric fields [57] . Another advantage of oxygen-free FL is that the technique offers process control that is superior to former FL techniques. The use of hard devices and the high-strength bonding method provides a considerable reduction of process timescales for channel relaxation, polymerization and flow. Also, the programmable sheath-like inert flows allow for on-the-fly alteration of particle height, a significant advantage over the current method in which particle height is dictated by channel height. Finally, oxygen-free FL greatly expands the library of synthesis materials that can be used, enabling the creation of particles from previously inaccessible reagents such as organic solvents. Through the fabrication of solvent compatible NOA81 devices, we synthesized new multifunctional particles from seven distinct organic precursors, including four monomers (PEGDA, TMPTA, PUA, and NOA), for supporting matrix and three nano-entities (ruthenium, QDs and SWNTs) for functional units. Also, we demonstrated the synthesis of NIR barcoded particles capable of label-free and real-time detection of analyte. Significantly, all functions of the barcoded particles work around the second NIR window, which greatly reduces the likelihood of signal interference from tissues, cells and biofluids in potential in-vivo multiplexed sensing applications. By allowing for a new range of synthesis conditions and environments, we believe that oxygen-free FL can be a powerful means to achieve novel categories of functional particles for diverse applications. Materials For swelling experiments, we used an organic solvent consisted of 98% (v/v) toluene (EMD Chemical) containing 2% (v/v) magnetic nanoparticles solution (EMG 905, Ferrotec, for visualization). PEG structures inside NOA devices were generated from a monomer solution containing 60% (v/v) PEGDA 700 (Sigma Aldrich), 10% (v/v) 2–hydroxy-2–methylpropiophenon (PI, Sigma Aldrich), and 30% (v/v) PEG 200 containing 20 mg ml −1 of red acrylate 13 (Sigma Aldrich). PEG particles encapsulating ruthenium were synthesized using solution of 84% (v/v) PEGDA 200 (Sigma Aldrich), 10% (v/v) PI, 1% (v/v) 1-vinyl-2-pyrrolidone (Sigma Aldrich), and 5% (v/v) ruthenium complex (II) dye solution. The dye solution was prepared by dissolving dichlorotris(1,10-phenanthroline) ruthenium (II) hydrate (Sigma Aldrich) powder into a mixture of methanol and toluene (4:1, v/v) at a concentration of 5 mg ml −1 . Other PEG particles were made of the composition as in Fig. 3a . Unless noted, PEG inert flows were PEG 200 (Sigma Aldrich) containing the same PI concentration as the accompanying monomer solution. In experiments to find the critical gel point of PEGDA 575, the monomer solutions consisted of 5% (v/v) PI, 1% (v/v) methacryloxyethyl thiocarbamoyl rhodamine B (Polysciences) in PEG 200 (1 mg ml −1 ), 4% (v/v) Food coloring (Tone Brothers), X % (v/v) PEGDA 575, and 90- X % (v/v) PEG 200. PUA and TMPTA (Polysciences) particles were prepared from a prepolymer composition of 55% (v/v) monomer, 35% (v/v) toluene and 10% (v/v) PI. The liquid PUA precursor (MINS 311RM) was kindly provided by Minuta Tech. For QDs stock solution, we purchased 915-nm CdTeSe/ZnS QDs dispersed in toluene at a concentration of 25 mg ml −1 (Nano Optical Materials). QDs monomer mixture consisted of 10 % (v/v) PI, 40% (v/v) NOA81 (Norland Products), and 50% QDs solution. The QDs concentration was adjusted by toluene dilution of stock solution. In the synthesis of NIR barcoded particles, the PEG probe region was made of 10 % (v/v) PI, 30 % (v/v) SWNT/PDDFs toluene solution, and 60% (v/v) PEGDA 700. To disperse SWNT in toluene, a 5-mg portion of SWNT was added into 10 ml of toluene containing PDDF (100 mg). The resulting mixture was then sonicated using a probe-tip sonicator for 90 min at 10 W in an ice bath. The SWNT solution was centrifuged for 40 min at 16,000 g , and then the supernatant was decanted for further experiments. Lastly, tergitol inert flows were tergitol NP-10 (Sigma Aldrich) containing 10% (v/v) PI. iCVD process All iCVD films were deposited in a custom built vacuum reactor (Sharon Vacuum) with a radius of 12 cm, as previously described [58] . The ChromAlloy filaments (Goodfellow) were mounted in a parallel array to provide the thermal excitation, heated by a DC power supply (Sorensen). The filament temperature was measured by a K-type thermocouple (Omega Engineering) attached to one of the filaments. The vertical distance between the filament and the deposition stage was 1.5 cm. The stage was back-cooled by a recirculating chiller/heater (NESLAB), which served as the purpose of maintaining the substrate temperature constant to prevent the heating of the sample owing to the heated filaments. All the chemical species were used as purchased, without further purification. tert-Butyl peroxide (Aldrich, 97%) initiator at room temperature, was fed into the reactor through a mass flow controller (model 1,479, MKS Instruments) at 1 sccm. iCVD deposition conditions utilizing the monomer 4-aminostyrene (4-AS) (Aldrich, 97%) and glycidyl methacrylate (GMA) (Aldrich, 97%) were adopted from previous work reported by Xu and Mao [35] , [59] . Total pressure in the vacuum chamber was maintained at 0.3 torr and 0.2 torr for 4-AS and GMA depositions, respectively. Nano-adhesive bonding process Poly(glycidyl methacrylate) and Poly(4-aminostyrene) films were deposited on the top and bottom NOA channels via iCVD, respectively. To finish the construction of the two-layer NOA device, the top channel was assembled on the bottom channel and the device was fully cured under vacuum at 90 °C for 24 h. The ring-opening curing reaction of epoxy with amine group can form a strong covalent bond between the two channels. Curing time was intentionally prolonged to 24 h to ensure bond formation. Stop flow lithography set-up The set-up for stop flow lithography (SFL) uses pressure provided by a compressed-air source to drive flow inside the microfluidic channels. The compressed-air flow control system is described in our previous work [39] . Devices were mounted on an inverted microscope (Axiovert 200, Zeiss) equipped with a VS25 shutter system (UniBlitz) to precisely control the ultraviolet exposure dose. A photomask was then inserted into the field-stop of the microscope. The masks were designed in AUTOCAD 2005 and printed using a high-resolution printer at CAD Art Services (Bandon, OR). A Lumen 200 (Prior Scientific) served as the source of ultraviolet light. A filter set that allowed wide ultraviolet excitation (11,000v2: UV, Chroma) was used to select light of the desired wavelength. The VS25 shutter system driven by a computer-controlled VMM-D1 shutter driver provided specified pulses of ultraviolet light. The shutter-mediated ultraviolet exposures were synchronized with the stop flow system, using Python, to allow the user to cycle SFL process automatically through the specification of a flow duration, a stoppage duration, and an exposure time. Typical exposure times used were 30–300 ms and pressures ranged from 0.05 to 15 psi. Hydrodynamic resistance measurement We developed a modified hydrodynamic resistance model to estimate volumetric flow rates from inlet pressures. In this approach, we control inlet pressures to generate the three meta-stable hydrodynamic states shown in Supplementary Fig. S6 . In the first step, we set up all inlet pressures to a fixed value, 2.0 psia. Then, we independently reduce P 2 and P 3 to satisfy each case. For the first case, we reduce both P 2 and P 3 to meet the moment at which flow colours are optically clear on intersections. As we use food colouring to distinguish flows, the moment stands for that volumetric flow rates, Q 2 and Q 3 are zero while Q 1 is non-zero. As shown in Supplementary Fig. S6a, Q 1 has no colour while Q 2 and Q 3 colours are red and green, respectively. In this meta-stable status, we can create a resistance diagram and successively set up two equations by mass conservation. The diagram and equations can be found next to the optical image in Supplementary Fig. S6a . For the other two cases ( Supplementary Figs S6b and S6c ), we can do the same process and eventually write six equations with known nine inlet pressures and R 4 . R 4 can be just estimated from channel geometry, as the resistance is not combined with inlets and corners. As the six equations have six unknown variables, we can determine all hydrodynamic resistances. Supplementary Table S3-S6 summarize specific inlet pressures satisfying each case and hydrodynamic resistance values extracted from the pressures. Near-infrared fluorescence imaging/spectrum analysis NIR-fluorescence spectra of SWNTs from barcoded particles were measured using a home-built NIR fluorescence microscope. Briefly, a Zeiss AxioVision inverted microscope was coupled to a Princeton Instruments InGaAs 1-D array detector through a PI-Acton SP 150 spectrograph. Samples were excited by a 785-nm laser at 30 mW and the emission from 900 to 1,400 nm was detected. Spectra were acquired for 2 s using a ×50 objective. Fluorescence images of particles were taken using a fluorescence microscope (Carl Zeiss, Axiovert 200), with a CCD camera (Carl Zeiss, ZxioCam MRm) and 2D InGaAs array (Princeton Instruments OMA 2D). Samples were excited by a 658-nm laser (LDM-OPT-A6-13, Newport Corporation) at 35 mW and the emission from 900 to 1,400 nm was detected for 1 s using a ×20 objective. For proton detection using a Janus particle, a particle was placed in the channel, which was mounted on the microscope stage. Then, a particle was focused using a ×50 objective to maximize its NIR fluorescence intensity. A diluted solution of HCl (70 μl, 7.2 M) was slowly added into the solution (140 μl) in the channel, and the NIR fluorescence response to protons was measured in real-time for 10 min (785-nm laser, 2 s of exposure time). How to cite this article: Bong, K. W. et al . Non-polydimethylsiloxane devices for oxygen-free flow lithography. Nat. Commun. 3:805 doi: 10.1038/ncomms1800 (2012).